Monolayer behaviour in bulk ReS2due to electronic and vibrational decoupling Semiconducting transition metal dichalcogenides consist of monolayers held together by weak forces where the layers are electronically and vibrationally coupled. Isolated monolayers show changes in electronic structure and lattice vibration energies, including a transition from indirect to direct bandgap. Here we present a new member of the family, rhenium disulphide (ReS 2 ), where such variation is absent and bulk behaves as electronically and vibrationally decoupled monolayers stacked together. From bulk to monolayers, ReS 2 remains direct bandgap and its Raman spectrum shows no dependence on the number of layers. Interlayer decoupling is further demonstrated by the insensitivity of the optical absorption and Raman spectrum to interlayer distance modulated by hydrostatic pressure. Theoretical calculations attribute the decoupling to Peierls distortion of the 1T structure of ReS 2 , which prevents ordered stacking and minimizes the interlayer overlap of wavefunctions. Such vanishing interlayer coupling enables probing of two-dimensional-like systems without the need for monolayers. Atomically thin monolayer transition metal dichalcogenides (sTMDs) are a new class of two-dimensional (2D) materials with the chemical formula MX 2 , where M is a transition metal (Mo, W and Re) and X is a chalcogen (S, Se and Te) element. Monolayer sTMDs are promising functional materials for next-generation flexible optoelectronics and photovoltaics applications owing to their mechanical flexibility, chemically and environmentally stability, optical properties and low operating voltages in various device configurations [1] , [2] , [3] . One of the landmark features of sTMDs is that they undergo a crossover from indirect bandgap in the bulk to direct bandgap in monolayers [4] , and as a result, monolayer sTMDs become direct-gap semiconductors that absorb and emit light efficiently. Currently, this crossover has been observed in all members of the sTMDs family known in the field, and is attributed to a strong interlayer coupling and explained as a confinement effect in the thickness direction. Here we present a new member of the sTMDs family, rhenium disulphide (ReS 2 ), in which the band renormalization is absent and the bulk behaves as electronically and vibrationally decoupled monolayers. Such unique response originates from lack of interlayer registry and weak interlayer coupling arising from Peierls distortion of the 1T structure of ReS 2 , as confirmed by high-resolution transmission electron microscopy (HRTEM), electron diffraction and density functional theory (DFT) calculations. Consequently, from bulk to monolayers, ReS 2 remains a direct-bandgap semiconductor, its photoluminescence (PL) intensity increases, whereas its Raman spectrum remains unchanged with increasing number of layers. Even after further modulating the interlayer distance (coupling) by external hydrostatic pressure, the optical absorption and Raman spectrum remain unchanged, implying that the interlayer interaction is indeed rather weak. The presented results establish ReS 2 as an unusual, new member of the sTMDs family where the bulk acts as if it is electronically and vibrationally monolayers. 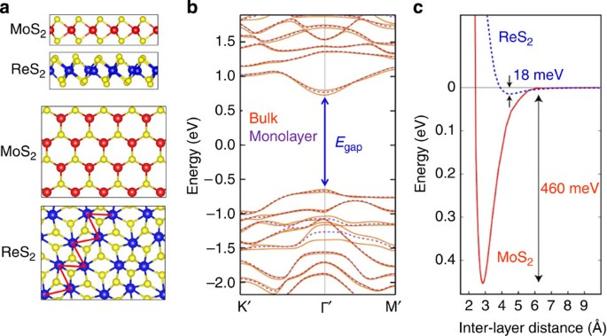Figure 1: Different crystal structure and band structure of ReS2from conventional sTMDs. (a) Side (top two panels) and top view (bottom two panels) of ReS2with distorted 1T crystal structure compared with the 1H structure of conventional sTMDs. The Re atoms dimerize as a result of the Peierls distortion forming a Re chain denoted by the red zigzag line. (b) DFT calculated electronic band structure of bulk (orange solid curves) and monolayer (purple dashed curves) ReS2. Both are predicted to be a direct bandgap semiconductor with nearly identical bandgap value at the Γ point. (c) The calculated total energy of the system as a function of interlayer separation. The significantly shallower depth of the well in ReS2implies much weaker interlayer coupling energy in ReS2as compared with MoS2. DFT calculations and calculated crystal structure Figure 1a shows a comparison of the structure of a single layer of ReS 2 with the conventional 1H structure of sTMDs such as MoS 2 . For ReS 2 , DFT calculations show that the hexagonal (H) phase is unstable, whereas the octahedral (T) phase goes through the Peierls distortion, resulting in buckled S layers and zigzag Re chains along one of the lattice vectors in the plane ( Fig. 1a bottom, Supplementary Fig. 1 ). The resultant lattice in Fig. 1a can be regarded as a distorted 1T structure ( Supplementary Notes 1 and 2 ). Owing to the reduced crystal symmetry, ReS 2 displays a more complex Raman spectrum than conventional sTMDs, as will be discussed later. DFT calculations reveal that bulk and monolayer ReS 2 have nearly identical band structures ( Fig. 1b ), both being direct-bandgap semiconductors with a predicted generalized gradient approximation (GGA) bandgap at E gap =1.35 eV (bulk) and 1.43 eV (monolayer), respectively ( Supplementary Note 3 ). This is in stark contrast to conventional sTMDs, where the band structure is strongly dependent on the number of layers [4] , [5] . Our DFT calculations ( Fig. 1c ) also show that adjacent layers in ReS 2 are indeed only weakly coupled to each other, with a coupling energy of~18 meV per unit cell, <8% of that of MoS 2 (460 meV for the corresponding 2 × 2 conventional cell). Figure 1: Different crystal structure and band structure of ReS 2 from conventional sTMDs. ( a ) Side (top two panels) and top view (bottom two panels) of ReS 2 with distorted 1T crystal structure compared with the 1H structure of conventional sTMDs. The Re atoms dimerize as a result of the Peierls distortion forming a Re chain denoted by the red zigzag line. ( b ) DFT calculated electronic band structure of bulk (orange solid curves) and monolayer (purple dashed curves) ReS 2 . Both are predicted to be a direct bandgap semiconductor with nearly identical bandgap value at the Γ point. ( c ) The calculated total energy of the system as a function of interlayer separation. The significantly shallower depth of the well in ReS 2 implies much weaker interlayer coupling energy in ReS 2 as compared with MoS 2 . Full size image HRTEM measurements and determination of crystal structure To study the structure and define the stacking order of ReS 2 , we deployed extensive HRTEM and electron diffractometry measurements. In Fig. 2a , we display the HRTEM image taken from two ReS 2 flakes, one with the layers perpendicular (red square) and the other parallel (green square) to the electron beam, confirming high crystallinity of the exfoliated ReS 2 . This arrangement is convenient as it provides a view of the crystalline structure from two orthogonal directions. Fast Fourier transform images taken perpendicular to the planes displays quasi-hexagonal pattern formed by (100), (001) and (110) reflections with the diffraction spot width defined by the beam convergence (~0.1 mrad) ( Fig. 2b top), consistent with a well-defined crystalline structure (simulated kinematic diffraction patterns in Fig. 2c top). To provide insight into the layer stacking order, we have oriented the crystal with the electron beam pointing at the [210] axis. The diffraction pattern consists of (10) and (002) reflections ( Fig. 2b,c bottom). The lack of odd ((001), (003), (005) and so on.) reflections suggests lack of specific (Bernal) stacking, unlike in 2H-MoS 2 that possesses Bernal stacking between the layers. The (0,0,2 l ) reflections are inhomogeneously broadened both in the 001 and (10) directions. Nano-beam electron diffraction pattern in Fig. 2d and inset allow direct comparison of the broadening because of the particular sample geometry. For simplicity, we attribute all the inhomogeneous broadening of the 0,0,2 l reflections to fluctuation in interlayer distance. From this analysis, the interlayer spacing is determined to vary between 6.0 and 6.9 Å. This reduced degree of crystallinity is not turbostratic in nature; rather, it is a consequence of weak interlayer bonding with small in-plane displacements from equilibrium position ( Supplementary Notes 1,2 and 7 ). 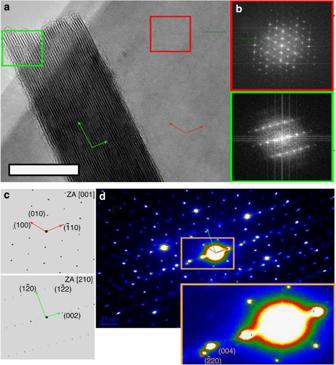Figure 2: Structural characterization of ReS2. (a) HRTEM images taken from ReS2along in- and out-of-plane directions. There are two flakes: one flake’s basal plane is perpendicular to the electron beam (red square box) and the other flake’s basal plane is oriented parallel to the beam (green square box). Scale bar, 20 nm. (b) Fast Fourier transform images from the denoted red/green windows. (c) Simulated kinematic diffraction patterns, and (d) nano-beam electron diffraction pattern. Inset: Zoom-in image to the nano-beam electron diffraction pattern. Figure 2: Structural characterization of ReS 2 . ( a ) HRTEM images taken from ReS 2 along in- and out-of-plane directions. There are two flakes: one flake’s basal plane is perpendicular to the electron beam (red square box) and the other flake’s basal plane is oriented parallel to the beam (green square box). Scale bar, 20 nm. ( b ) Fast Fourier transform images from the denoted red/green windows. ( c ) Simulated kinematic diffraction patterns, and ( d ) nano-beam electron diffraction pattern. Inset: Zoom-in image to the nano-beam electron diffraction pattern. Full size image Comparison between PL behaviour of ReS 2 versus other sTMDs Considering such contrast in the crystal structure, we next focus experimentally on the physical properties of ReS 2 flakes. Mono- and multilayer ReS 2 were mechanically exfoliated from synthetic bulk crystals (see Methods section for crystal growth) onto Si substrates with 90 nm thermal oxide [6] . These ReS 2 flakes were characterized using atomic force microscopy (AFM), Raman spectroscopy, micro-PL (μPL), and nano-Auger electron spectroscopy (AES). Nano-AES elemental composition analysis revealed an S/Re ratio of 1.98±0.10 ( Supplementary Fig. 8 , Supplementary Note 6 ). Tapping-mode AFM scan typically yielded 0.7 nm thickness for the monolayers. For comparison, monolayers and multilayers of conventional sTMDs (MoS 2 , MoSe 2 , WSe 2 and WS 2 ) were also prepared by mechanical exfoliation from bulk crystals. All ReS 2 flakes exhibit μPL at room temperature with a peak in the range of 1.5–1.6 eV. The peak energy increases slightly (by <10%) for an isolated monolayer ( Fig. 3a ). The integrated PL intensity increases with the number of layers, and starts to saturate for flakes thicker than six layers, as shown in Fig. 3b . This is in stark contrast to the behaviour observed in conventional sTMDs such as MoS 2 (ref. 4 ), MoSe 2 (ref. 7 ), WS 2 and WSe 2 (ref. 8 ), where the monolayer PL intensity is enhanced by orders of magnitude as a result of the crossover from an indirect bandgap in the bulk to a direct bandgap in monolayers. In those Mo and W systems, the PL in the indirect-bandgap multilayers arises from hot luminescence [4] across the wider direct bandgap, and is exponentially weaker in thicker layers. In addition, the PL peak position of these conventional sTMDs increases drastically by 30–60% for thinner layers ( Fig. 3c ), which can be explained by stronger out-of-plane quantum confinement with decreasing thickness [4] . In contrast, the PL peak of ReS 2 is nearly independent of the number of layers, indicating that thinning down the flake does not enhance the quantum confinement of electrons in the system, and that neighbouring monolayers in the flake are already largely electronically decoupled. 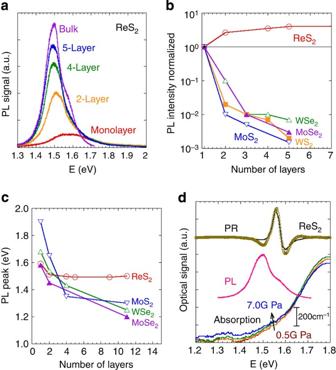Figure 3: Optical properties of ReS2in comparison with conventional sTMDs. (a) PL spectrum of ReS2flakes with different number of layers. (b) Integrated PL intensity as a function of number of layers (normalized to that of monolayer) in ReS2, MoS2, MoSe2, WS2and WSe2. (c) Change in the PL peak position as a function of number of layers in ReS2, MoS2,MoSe2and WSe2. (d) Absorption coefficient of a bulk ReS2flake (thickness ~10 μm) at hydrostatic pressures ranging from 0.5 to 7.0 GPa. Also shown is the PL and photo-modulated reflectance spectra of bulk ReS2taken at ambient condition. It can be seen that a direct bandgap exists at 1.55±0.05 eV and is insensitive to the pressure. Figure 3: Optical properties of ReS 2 in comparison with conventional sTMDs. ( a ) PL spectrum of ReS 2 flakes with different number of layers. ( b ) Integrated PL intensity as a function of number of layers (normalized to that of monolayer) in ReS 2 , MoS 2 , MoSe 2 , WS 2 and WSe 2 . ( c ) Change in the PL peak position as a function of number of layers in ReS 2 , MoS 2, MoSe 2 and WSe 2 . ( d ) Absorption coefficient of a bulk ReS 2 flake (thickness ~10 μm) at hydrostatic pressures ranging from 0.5 to 7.0 GPa. Also shown is the PL and photo-modulated reflectance spectra of bulk ReS 2 taken at ambient condition. It can be seen that a direct bandgap exists at 1.55±0.05 eV and is insensitive to the pressure. Full size image Electronic decoupling in ReS 2 To further test the interlayer decoupling in ReS 2 , we modulate its interlayer distance by applying hydrostatic pressure using a diamond anvil cell (DAC). The hydrostatic pressure is applied via a liquid medium onto a bulk flake (~10 μm), where the pressure is calibrated with the standard Ruby luminescence [9] ( Supplementary Note 5 ). The transparent DAC window allows experiments for micro-Raman and optical micro-absorption. Comparing the absorption curves with the PL and photo-modulated reflectance (see Supplementary Fig. 7 , Supplementary Note 5 ) spectra in Fig. 3d , the bandgap of ReS 2 is determined to be E gap =1.55 eV, close to the DFT calculated E gap . In Fig. 3d , the optical absorption curve shows nearly no change under the application of hydrostatic pressure up to 7 GPa. The out-of-plane linear elastic moduli of ReS 2 and MoS 2 are estimated to be 0.4 and 20 GPa, respectively, calculated from the second derivative of the interlayer coupling energy in Fig. 1c . Therefore, a pressure of 7 GPa would significantly reduce their interlayer distance. In bulk MoS 2 where adjacent layers are coupled, the pressure dependence of the bandgap is d E gap /d P ~0.02 eV per GPa (refs 10 , 11 ), corresponding to a 0.14-eV shift of the absorption edge for the pressure range in Fig. 3d , whereas ReS 2 shows a total shift of 0.04 eV at the most. Therefore, the overlap of electron wavefunctions from adjacent layers is much weaker in ReS 2 than in MoS 2 , such that a modulation of the interlayer distance cannot renormalize the band structure in the former. Vibrational decoupling in ReS 2 The much weaker interlayer interaction energy shown in Fig. 1c also leads to a decoupling of lattice vibrations between adjacent layers in ReS 2 . In Fig. 4a,b , we compare calculated phonon dispersion with the measured Raman spectrum of monolayer ReS 2 . The Raman spectrum displays at least 11 modes in the 100–400 cm −1 range, which is significantly more than for sTMDs with higher crystal symmetries. These Raman peaks are mostly caused by the low crystal symmetry and are associated with fundamental Raman modes (A 1g , E 2g , and E 1g ) coupled to each other and to acoustic phonons. The two most prominent Raman peaks are at 163 and 213 cm −1 , respectively, and correspond to the in-plane (E 2g ) and mostly out-of-plane (A 1g -like) vibration modes ( Supplementary Fig. 6 , Supplementary Note 3 ). Comparison between the Raman spectra of monolayer and bulk ReS 2 ( Fig. 4c ) does not show detectable changes within the 0.3 cm −1 resolution. Again in contrast, the Raman spectrum is known to be highly sensitive to the number of layers in MoS 2 ( Fig. 4d ) and other sTMDs [12] , [13] , [14] . For example, going from the bulk to monolayer sTMDs, the E 2g mode in MoS 2 typically stiffens by ~5 cm −1 , and the A 1g mode typically softens by a similar amount. As ReS 2 is vibrationally decoupled, its Raman spectrum is expected to be also less sensitive to hydrostatic pressure compared with other sTMDs. In Fig. 5a , we present the pressure induced change in the most prominent Raman peaks for bulk ReS 2 and MoS 2 . As the interlayer coupling directly affects the out-of-plane vibration modes, we focus on the pressure behaviour of the Raman peaks associated with the out-of-plane vibration. The primarily out-of-plane, A g -like Raman peak in ReS 2 located at 213 cm −1 stiffens by only ~1 cm −1 per GPa of hydrostatic pressure, whereas it is >2.7 cm −1 per GPa for the A g mode in MoS 2 , 2.2 cm −1 per GPa in MoSe 2 and 2.5 cm −1 per GPa in MoTe 2 (ref. 15 ). In Fig. 5b , these numbers are compared against each other. Because the 213 cm −1 vibration mode in ReS 2 is not purely A g , but mixed with the more pressure-sensitive, in-plane E g mode (see Supplementary Note 3 ), the intrinsic pressure coefficient of the A g mode is expected to be even lower in ReS 2 . Moreover, considering the ~50 times lower elastic modulus of ReS 2 than MoS 2 , the deformation coefficient (dA g /d z , where z is interlayer distance) of out-of-plane vibration in ReS 2 is estimated to be orders of magnitude lower than MoS 2 . Related to the observed electronic and vibrational decoupling in ReS 2 , the out-of-plane thermal conductivity is also calculated and found to be much smaller than that of MoS 2 (κ MML:MoS 2 ⊥ / κ ReS 2 ⊥ ≈ 42 ) , whereas the in-plane thermal conductivity of ReS 2 and MoS 2 are on the same order of magnitude ( Supplementary Note 4 ). 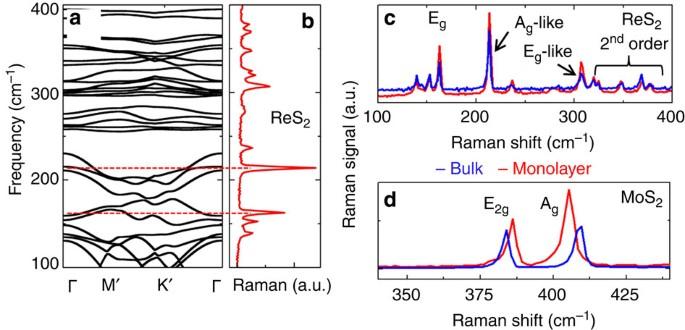Figure 4: Vibrational properties of ReS2and Raman spectra. (a) Calculated phonon dispersion for monolayer ReS2. The phonon dispersion of bulk ReS2(Supplementary Fig. 6) remains nearly identical to that of monolayer. (b) Raman spectrum measured on a monolayer ReS2. (c) Raman spectrum taken on bulk (blue) and monolayer (red) ReS2. (d) Same on MoS2.The Raman spectrum of ReS2shows no thickness dependence, whereas the MoS2in-plane (E2g) and out-of-plane (A1g) peaks are highly sensitive to the number of layers. Figure 4: Vibrational properties of ReS 2 and Raman spectra. ( a ) Calculated phonon dispersion for monolayer ReS 2 . The phonon dispersion of bulk ReS 2 ( Supplementary Fig. 6 ) remains nearly identical to that of monolayer. ( b ) Raman spectrum measured on a monolayer ReS 2 . ( c ) Raman spectrum taken on bulk (blue) and monolayer (red) ReS 2 . ( d ) Same on MoS 2. The Raman spectrum of ReS 2 shows no thickness dependence, whereas the MoS 2 in-plane (E 2g ) and out-of-plane (A 1g ) peaks are highly sensitive to the number of layers. 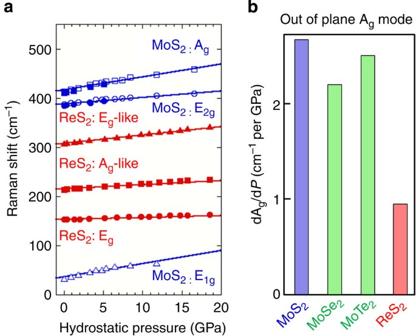Figure 5: Pressure dependence of Raman peaks of ReS2compared with MoS2. (a) Variation of the most prominent Raman peaks of bulk ReS2and MoS2as a function of applied hydrostatic pressure. Empty blue points are taken from ref.15, and filled red and blue points are from this work. The pressure dependence of MoS2Agand E2gpeaks is confirmed by the good agreement between this work and ref.15. The straight lines are linear fit to the experimental data. (b) Comparison of pressure coefficient (dAg/dP) of the out-of-plane (Ag) Raman peaks of MoS2, MoSe2, MoTe2and ReS2. It can be seen that the ReS2out-of-plane vibration shows at least a factor of 2 weaker dependence on pressure. Full size image Figure 5: Pressure dependence of Raman peaks of ReS 2 compared with MoS 2 . ( a ) Variation of the most prominent Raman peaks of bulk ReS 2 and MoS 2 as a function of applied hydrostatic pressure. Empty blue points are taken from ref. 15 , and filled red and blue points are from this work. The pressure dependence of MoS 2 A g and E 2g peaks is confirmed by the good agreement between this work and ref. 15 . The straight lines are linear fit to the experimental data. ( b ) Comparison of pressure coefficient (dA g /d P ) of the out-of-plane (A g ) Raman peaks of MoS 2 , MoSe 2 , MoTe 2 and ReS 2 . It can be seen that the ReS 2 out-of-plane vibration shows at least a factor of 2 weaker dependence on pressure. Full size image On the basis of the distorted crystal structure, we discuss the physical origin of the vanishing interlayer coupling in ReS 2 . We first note that each Re atom has seven valence electrons and therefore has one extra electron in the 1T or H structure. DFT calculations show that when this electron contributes to the formation of Re–Re bonds, the total energy of the system is lowered, the Eigen values of the acoustic phonons become real and the lattice becomes a distorted 1T structure as shown in Fig. 1a ( Supplementary Notes 1 and 2 ). Upon transition from 1T (1H) to the distorted 1T structure, the energy gain is 1.1 (0.9) eV per ReS 2 molecule. In the distorted 1T structure, the Re atoms in the layer dimerize in such a way that they form a zigzag Re–Re chain extending along one of the lattice vectors [16] , [17] . Interestingly, by geometry consideration, the presence of the Re chains eliminates the energy benefit for the ReS 2 layers to order in Bernal (AB) or rhombohedral (ABC) stacking that occurs in other sTMDs. Our DFT calculations show that while sliding one MoS 2 monolayer over the other, one yields variation in total energy of ~200 meV; for ReS 2 the energy difference is just on the order of 5 meV ( Supplementary Note 2 ). The lack of ordered stacking significantly reduces the interlayer coupling energy, akin to turbostratic graphite where the interlayer interaction is significantly weaker than that of Bernal-stacked graphite. Another factor contributing to the vanishing interlayer coupling comes from a much weaker polarization inside the ReS 2 layers. Our charge density calculations show that, compared with MoS 2 , there is a smaller charge difference between the neighbouring Re and S planes, and hence a smaller dipole moment residing in each layer. As a result of the weak intra-layer polarization, the van der Waals force and the binding energy between adjacent ReS 2 layers are very weak ( Supplementary Fig. 4 ). Therefore, ReS 2 bulk crystals would be an ideal platform to probe 2D excitonic and lattice physics, circumventing the challenge of preparing large-area, single-crystal monolayers. Experiments on 2D systems that are currently limited by the availability of large-area monolayers or by low sensitivity to monolayer thickness would become possible on the bulk ReS 2 . In this sense, the presented results introduce a new type of sTMDs with distinct physical properties from conventional members of the sTMDs explored to date. Micro-Raman and μPL experiments Raman and PL measurements were performed using a × 100 objective in a Renishaw micro-Raman/PL system. The excitation laser wavelength is 488 nm, with laser power ranging from 100 to 1,000 μW power on a ~6-μm 2 spot. DAC measurements Two symmetric DACs with type II diamonds of 300 and 500 μm flat culets were utilized for Raman and optical absorption experiments, respectively. The pressure volume of 120 μm in height and 70 μm in diameter was machined from a 250-μm-thick stainless steel gaskets. A methanol–ethanol mixture of 4:1 volume ratio was used as a pressure transmitting medium. Hydrostatic pressure applied inside the chamber hole was calibrated by measuring the R1 PL line shift of ruby. A series of Raman spectra were taken on a ReS 2 single-crystal flake at various pressures up to 26 GPa using a × 50 magnification, 18-mm working distance objective, on the Renishaw micro-Raman/PL system. For optical absorption measurements with the DAC, a home-built optics system equipped with a 0.5-m single-grating monochromator and a tungsten–halogen lamp was used. The sample flake was magnified and imaged on the focal plane, where an apertured silicon photodiode detects the light intensity with a lock-in amplifier. ReS 2 growth Single crystals of ReS 2 were grown by the chemical vapour transport method, using Br 2 as a transport agent, leading to n-type conductivity. Before the crystal growth, quartz tubes containing Br 2 and the reacting elements (Re: 99.95% pure, S: 99.999%) were evacuated and sealed. The quartz tube was placed in a three-zone furnace and the charge pre-reacted for 24 h at 800 °C with the growth zone at 1,000 °C, thereby preventing transport of the product. The furnace was then equilibrated to give a constant temperature across the reaction tube and was programmed over 24 h to produce the temperature gradient at which single-crystal growth takes place. The best results were obtained with a temperature gradient of 1,060 to 1,100 °C. High-resolution TEM HRTEM and diffractometry was performed on JEOL2100F microscope equipped with EDS and EELS spectrometers. The exfoliated ReS 2 was transferred to electron transparent supports (C-flat carbon support and patterned SiN membranes from EMS). A number of 20–50-nm-thick ReS 2 crystals were studied in various orientations including the in-plane and out-of-plane configurations. DFT calculations Structural, electronic and vibrational properties have been calculated using GGA-PBE (Perdew-Burke-Ernzerhof) functional, as implemented in the VASP code [18] , [19] within the DFT, which is demonstrated to yield rather accurate results for sTMDs. Calculations were performed using the Generalized Gradient Approximation [20] and projector augmented-wave potentials [21] . The kinetic energy cutoff for the plane-wave basis set was 500 eV. In the self-consistent potential and total energy calculations of ReS 2 layers, a set of (31 × 31 × 1) k-point samplings was used for Brillouin zone integration. The convergence criterion of self-consistent calculations for ionic relaxations was 10 −5 eV between two consecutive steps. By using the conjugate gradient method, all atomic positions and unit cells were optimized until the atomic forces were <0.01 eV/Å. Pressures on the lattice unit cell were decreased to values <0.5 kbar. Phonon dispersion curves were obtained using the small displacement method [22] . How to cite this article: Tongay, S. et al. Monolayer behaviour in bulk ReS 2 due to electronic and vibrational decoupling. Nat. Commun. 5:3252 doi: 10.1038/ncomms4252 (2014).